Silicon isotopes indicate enhanced carbon export efficiency in the North Atlantic during deglaciation Today’s Sargasso Sea is nutrient starved, except for episodic upwelling events caused by wind-driven winter mixing and eddies. Enhanced diatom opal burial in Sargasso Sea sediments indicates that silicic acid, a limiting nutrient today, may have been more available in subsurface waters during Heinrich Stadials, millennial-scale climate perturbations of the last glacial and deglaciation. Here we use the geochemistry of opal-forming organisms from different water depths to demonstrate changes in silicic acid supply and utilization during the most recent Heinrich Stadial. We suggest that during the early phase (17.5–18 ka), wind-driven upwelling replenished silicic acid to the subsurface, resulting in low Si utilization. By 17 ka, stratification reduced the surface silicic acid supply leading to increased Si utilization efficiency. This abrupt shift in Si cycling would have contributed to high regional carbon export efficiency during the recent Heinrich Stadial, despite being a period of increasing atmospheric CO 2 . In the modern ocean, the North Atlantic subtropical gyre is classified as oligotrophic, with low surface nutrient concentrations and low annual primary productivity [1] . The Sargasso Sea, situated within the gyre, experiences a spring plankton bloom—despite being chronically Si limited [1] —as a result of seasonal wind-driven deep mixing from the upper boundary of the main thermocline ( Fig. 1 ). However, the deep supply of nutrients supports a bloom that represents only a transient phytoplankton standing stock concentrated in a deep (~100 m) chlorophyll a maximum of up to ~0.5 mg m −3 , a modest amount compared with regions of the open Southern Ocean (~1 mg m −3 ) and major upwelling zones and coastal areas (over 10 mg m −3 (ref. 2 )). In the Sargasso Sea, diatoms contribute strongly to export production, despite a significant proportion of primary productivity originating from smaller phytoplankton cells, as a result of a strong microbial loop [1] . There have been substantial efforts in the last decade to understand the impact of nutrient upwelling driven by cyclonic and Mode-Water mesoscale eddies on modern ecology, the latter of which promotes the growth of larger-sized phytoplankton (diatoms and dinoflagellates) [3] , but the role of these mesoscale processes in past carbon cycling and their potential impact on future global change remains unclear. 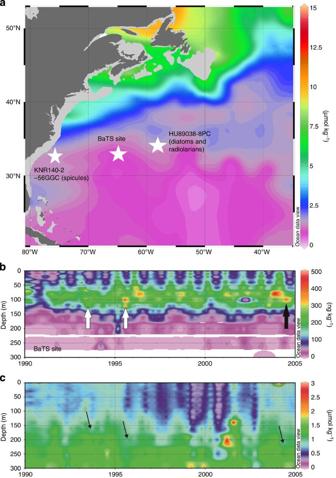Figure 1: Map showing the key localities for this study. (a) The stars show the localities of the Bermuda Time Series (BaTS) site, and new sediment core records discussed in this study. Note that OCE326-GGC5 was collected from the Bermuda Rise, very near the same location as HU89038-8PC. The colour contours show the concentration of Si(OH)4in μmol kg−1at 100 m, created using data from ref.10and Ocean Data View (version 4). (b) Chlorophylladata from the BaTS site from 1990 to 2005. The white arrows show documented eddies from the BaTS site3, and the black arrow shows a documented cold core ring during the EDDIES cruises55: (c) Si(OH)4concentrations at the BaTS site from 1990 to 2005, with arrows showing the drawdown of upwelled Si(OH)4due to biological uptake (note different scale toa); all data are from ref.60. Figure 1: Map showing the key localities for this study. ( a ) The stars show the localities of the Bermuda Time Series (BaTS) site, and new sediment core records discussed in this study. Note that OCE326-GGC5 was collected from the Bermuda Rise, very near the same location as HU89038-8PC. The colour contours show the concentration of Si(OH) 4 in μmol kg −1 at 100 m, created using data from ref. 10 and Ocean Data View (version 4). ( b ) Chlorophyll a data from the BaTS site from 1990 to 2005. The white arrows show documented eddies from the BaTS site [3] , and the black arrow shows a documented cold core ring during the EDDIES cruises [55] : ( c ) Si(OH) 4 concentrations at the BaTS site from 1990 to 2005, with arrows showing the drawdown of upwelled Si(OH) 4 due to biological uptake (note different scale to a ); all data are from ref. 60 . Full size image Multiproxy evidence points towards a widespread increase in supply of silicic acid (Si(OH) 4 )-rich waters during the abrupt climatic events of the last glacial and deglacial, including the Southern Ocean [4] , equatorial regions [5] and major coastal upwelling zones [6] . Sedimentary evidence also points towards anomalous and prolonged diatom blooms in the North Atlantic during abrupt events of the deglacial [7] , [8] , which would have had a significant impact on carbon cycling in the otherwise oligotrophic gyre. During the last glacial and deglaciation, abrupt millennial-scale Heinrich Stadials (HS) associated with iceberg-rafting events in the North Atlantic led to widespread and rapid reorganization of ocean circulation, which in turn resulted in shifts in heat transport, atmospheric pCO 2 and the supply of southern component water and nutrients to northern latitudes [9] . Southern component water plays an important role in the supply of essential nutrients such as Si(OH) 4 , which feeds the diatom growth that contributes significantly to marine carbon export production in the world’s oceans. Antarctic bottom water, formed by deep convection around Antarctica, contains high levels of macronutrients including Si(OH) 4 (>100 μM (ref. 10 )). Antarctic intermediate water (AAIW), formed by the subduction of cold, fresh surface waters near the polar front, has lower Si(OH) 4 concentrations (<70 μM, generally ~40 μM north of 20°S) compared with other nutrients (nitrate and phosphate) as a result of efficient uptake of Si by diatoms in the Southern Ocean [11] , and can influence the nutrient content of the thermocline in the South Atlantic by mixing across density surfaces [12] . There has been recent debate regarding the degree to which AAIW extent and composition fundamentally changed during the millennial-scale climate events of the late glacial/deglacial, the role played by wind-driven versus oceanographic processes in these changes, and the impact of these changes on diatom productivity (reviewed by ref. 8 ). Neodymium isotope evidence points both towards a volumetric increase in AAIW at intermediate depths of the equatorial regions [13] , [14] but also to a decline in AAIW in the Florida Straits during HS1 (ref. 15 ). While nutrient proxies cannot determine the origins of the water, they do indicate that the mid-depths of the South Atlantic were more enriched in Si(OH) 4 relative to other nutrients during HS1 than they are today [16] , [17] , suggestive of a northwards advance of AAIW into the North Atlantic during HS1 (ref. 18 ). Although there is evidence for increased diatom opal burial in the oligotrophic North Atlantic during Stadials [7] , there has been, as of yet, no quantified study of low-latitude silicon cycling during millennial-scale climatic change and its impact on carbon cycling. Here we use the silicon isotope composition of different opal-forming organisms, extracted from a sediment core in the Sargasso Sea (Bermuda Rise), which dwell at different depths in the water column, to reconstruct changes in Si cycling during the last deglaciation. Our results show that there were abrupt shifts in Si supply and utilization during this period, consistent with changes in oceanic stratification, which would have contributed to high regional carbon export efficiency. Opal-producing organisms in the Sargasso Sea sediment core Core HU89038-PC8 on the Bermuda Rise (33.7 °N, 57.6 °W, 3.5 km water depth) contains a notable opal-rich section radiocarbon dated to HS1 (from 330 to 500 cm depth or 16.5–18.6 calibrated ka) [19] . The sand-sized fraction of the opal-rich layer comprises 60±10% opal, and is dominated (~95%) by fragments of the large diatom Ethmodiscus rex (Rattray) Hendey, with radiolarians (including polycystine radiolarians), smaller diatoms and rare sponge spicules. E. rex are relatively deep dwelling, occupying a distinct niche by opportunistically migrating deeper (>100 m) by varying their cellular buoyancy to take advantage of deep nutrient supplies, and are found today in the oligotrophic gyre of the North Pacific in highly stratified waters away from major convergence zones [20] . E. rex cells subsequently undergo mass sinking at frontal zones or when stratification is broken by another physical mechanism, such as storm mixing [21] . Most polycystine radiolarians live in water depths of less than 250 m and this is especially true for large open-structure Spumellaria, which often have associated with them symbiotic algae (zooxanthellae) and must spend at least some time in the euphotic zone to survive. The most common radiolarians picked from the sediments in this study (see Methods) have all been recovered from depths between 100 and 390 m in the modern. The information available suggests that most, if not all, of the large Spumellaria analysed spent most of their lives in waters shallower than 250 m and possibly less than 100 m. While the presence of the E. rex layer in HU89038-PC3 is in itself suggestive of an unusual and prolonged shift in biogeochemical cycling during HS1, we can also quantify the silicon biogeochemical system using the silicon isotope composition of different siliceous plankton opal that live at different depths in the water column. The silicon isotope ratio ( δ 30 Si) of diatoms can be used as a measure of Si utilization in ambient seawater because preferential uptake of the lighter isotope of Si leads to progressive enrichment in the heavier isotopes [22] . Diatom material was sufficiently abundant in this section of HU89038-PC8 such that it was possible to hand-pick monospecific samples of E. rex and mixed samples of polycystine radiolarians, mostly large Spumellaria, for silicon isotope analysis (see Methods). The E. rex δ 30 Si ranged from +0.20 to +1.14‰ and the mixed Spumellaria radiolarian δ 30 Si ranged from +0.73 to +2.00‰ ( Supplementary Table 1 ). Spicule record from the Carolina Slope Our new diatom and radiolarian silicon isotope records provide information on the utilization of Si in surface waters of the Sargasso Sea, but an integrated view of a biogeochemical system relies on the robust quantification of inputs and outputs of essential nutrients, in this case Si(OH) 4 . Mid-depth benthic Si(OH) 4 concentrations of waters feeding the North Atlantic subtropical gyre were reconstructed using the δ 30 Si composition of abundant and well-preserved sponge spicules extracted from marine sediment core KNR140-2-56GGC from the Carolina Slope (32°56.3′N, 76°17.7′W; 1,400 m; Fig. 1 ). The δ 30 Si of seafloor-dwelling sponges has been shown to be a proxy for deep water Si(OH) 4 concentrations as a result of enhanced uptake and associated fractionation of Si under higher Si(OH) 4 concentrations [23] . Downcore sponge spicule δ 30 Si from KNR140-2-56GGC ranged from −1.22 to −1.93‰ ( Fig. 2 ; Supplementary Figs 1 and 2 ). The average δ 30 Si value of the Holocene (<10 ka, 0–400 cm) spicules extracted from KNR140-2-56GGC was significantly heavier (1 s.d.) than that of samples deeper than 400 cm (>10 ka), signifying that the sponges growing in the Holocene experienced lower ambient Si(OH) 4 conditions, on average, than sponges growing in the late glacial and deglacial ( Fig. 2 ; Supplementary Fig. 1 ). The modern core-top δ 30 Si value corresponds to ambient Si(OH) 4 concentrations of ~15–20 μM (ref. 10 ), matching modern observations at these depths and indicating a minimal impact of downslope transport on the spicule proxy. The mean Holocene value of spicule δ 30 Si corresponds to a Si(OH) 4 concentration of ~25 μM ( Fig. 2 ). Our record shows lighter δ 30 Si values, and therefore a higher Si(OH) 4 concentration (30–37 μM), corresponding to HS1 (~15–18 ka). Today, the core is bathed in North Atlantic Deep Water (NADW), and proxy-based reconstructions suggest intermediate depth waters of the North Atlantic were bathed in Glacial North Atlantic intermediate water (GNAIW) during the glacial [24] . Physical and chemical properties of North Atlantic sediment cores indicate that there was a weakening of GNAIW flow during HS1 (ref. 25 ), stagnation of intermediate waters and a shoaling of southern-sourced abyssal water [8] to within ~1,000 m water depth of our core site [26] . Alternatively, it is possible that the higher Si(OH) 4 concentrations at our core site during HS1 were a result of northwards flow of AAIW. The higher concentration of Si(OH) 4 supplying the intermediate depths of the North Atlantic during millennial-scale climate events is similar in magnitude to a previous reconstruction of South Atlantic intermediate depth Si(OH) 4 concentrations, and is consistent with cross-equator flow of southern-sourced waters into the North Atlantic during HS1 (ref. 17 ). Sedimentological properties of cores from the Carolina Slope indicate that the upper boundary of the GNAIW may have been deeper than 1,400 m before the Holocene, as indicated by a low content of red material that characterized sediments from the Labrador Sea ( Supplementary Fig. 3 , (ref. 27 )). Furthermore, the increase in Si(OH) 4 recorded at our core site is relatively modest, and reflects concentrations more typical of AAIW (<70 μM) rather than Antarctic bottom water (>100 μM). 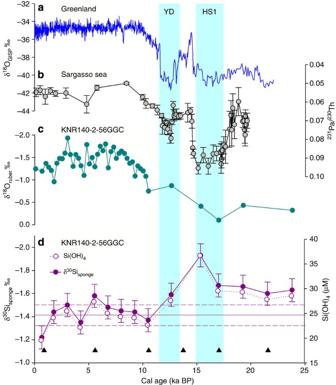Figure 2: Results from sediment core KNR140-2-56GGC. (a) Greenland ice core record ofδ18O (ref.61,b) marine sediment231Pa/230Th from the Bermuda Rise10,62and (c)δ18O ofGlobigerinides ruberfrom KNR140-2-56GGC27. (d) The silicon isotope composition of the sponge spicules plotted against age from 0 to 25 ka (solid symbols and lines), together with the reconstructed Si(OH)4concentration for core KNR140-2-56GGC (hollow symbols, dotted lines), calculated assuming [Si(OH)4]=270/(Δδ30Si+6.54)−53 (ref.23) where Δδ30Si is the difference in isotopic composition of the sponge spicules and seawater and assumingδ30Si(OH)4of dissolved silicon in seawater is +1.6‰. The purple line shows the mean Holocene spiculeδ30Si (solid) and 1σs.d. (dashed). All error bars show ±2σs.d. unless stated otherwise. The triangles show radiocarbon tie points (Supplementary Table 2). Vertical cyan bars show YD, younger Dryas; HS1, Heinrich Stadial one. Figure 2: Results from sediment core KNR140-2-56GGC. ( a ) Greenland ice core record of δ 18 O (ref. 61 , b ) marine sediment 231 Pa/ 230 Th from the Bermuda Rise [10] , [62] and ( c ) δ 18 O of Globigerinides ruber from KNR140-2-56GGC [27] . ( d ) The silicon isotope composition of the sponge spicules plotted against age from 0 to 25 ka (solid symbols and lines), together with the reconstructed Si(OH) 4 concentration for core KNR140-2-56GGC (hollow symbols, dotted lines), calculated assuming [Si(OH)4]=270/(Δ δ 30 Si+6.54)−53 (ref. 23 ) where Δ δ 30 Si is the difference in isotopic composition of the sponge spicules and seawater and assuming δ 30 Si(OH) 4 of dissolved silicon in seawater is +1.6‰. The purple line shows the mean Holocene spicule δ 30 Si (solid) and 1 σ s.d. (dashed). All error bars show ±2 σ s.d. unless stated otherwise. The triangles show radiocarbon tie points ( Supplementary Table 2 ). Vertical cyan bars show YD, younger Dryas; HS1, Heinrich Stadial one. Full size image Modelling the silicon cycle in the Sargasso Sea To quantify the efficiency of surface utilization of Si(OH) 4 in the Sargasso Sea using core material from HU89038-8PC, it is necessary to quantify the silicon isotope fractionation by both E. rex and Spumellarian radiolarians. Laboratory culture studies of diatoms of other genera indicate a mean fractionation of −1.1‰ (ref. 22 ) and show some limited evidence for variation with species and growth rate [28] . Although they may represent specific growth conditions, by using a monospecific sample in this study we have eliminated biases resulting from changing diatom assemblage over time and have quantified Si uptake by the likely dominant species ( E. rex representing ~95% of the opal fossils present in the HS1 layer). Measurements of δ 30 Si on the >63 μ opal fraction matched the E. rex within error, demonstrating that E. rex probably dominated opal production during this interval. The radiolarians in core HU89038-PC8 have a highly enriched δ 30 Si signal ( Fig. 3 ). Assigning a fractionation factor of −1.1‰, we can model the utilization by E. rex using isotope fractionation equations [29] , which yields a resulting water Si isotope composition of approximately +2.3‰ (from ~18 ka before present or BP) to +3‰ (from ~16.5 ka BP) and a radiolarian fractionation factor of approximately −1 to −2‰, consistent with the limited previous data (see Methods) [30] . If the two groups were growing from the same unaltered seawater (intermediate depth North Atlantic water or AAIW both have a δ 30 Si(OH) 4 of approximately +1.6‰, see Methods), the radiolarians would be positively discriminating against the lighter isotope of silicon during some time periods (for example, ~17 ka BP), which is not known in any biological system. This separation of radiolarian and diatom Si uptake could have occurred if either the radiolarians and diatoms are growing in a similar water mass but E. rex take up the silicon sufficiently rapidly such that they control the silicon chemistry of the seawater, or the radiolarians are not growing at the same depth as the E. rex cells. Either mechanism would imply that the radiolarians grew in water already isotopically enriched by E. rex. The radiolarian δ 30 Si signal also showed less variability than the E. rex signal, possibly because of temporal or spatial averaging over a season or different depths as a result of the mixed assemblage of radiolarians used for analysis. 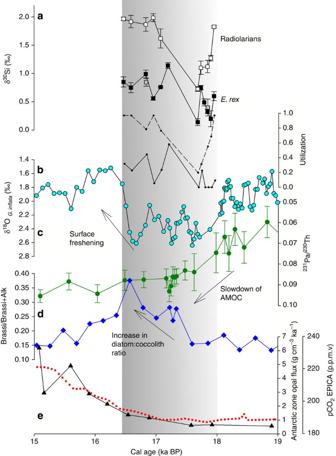Figure 3: Results from sediment core HU89038-8PC. (a) Silicon isotope results from sediment core HU89038-8PC (error bars show ±2σs.d.). The solid squares showδ30Si ofEthmodiscus rexdiatoms; the hollow squares showδ30Si of Spumellarian radiolarians; the grey squares showδ30Si of >63 μm opal. There is a positive correlation between theE. rexand radiolarianδ30Si measurements (Pearson’s correlation coefficientR=+0.71,n=10,P=0.02). The >63 μm opalδ30Si matched theE. rexopalδ30Si from the same depth within error, which would be expected, given thatE. rexconstituted over 95% of the bulk opal. The lines show calculated utilization of Si by theE. rex(solid line) and radiolarian (dashed line) cells, using a fractionation factor of −1.1‰ for theE. rex. We plot the mean utilization calculated for radiolarians with fractionation factors ranging from −0.9 to −2.1‰ (Methods). (b) The cyan circles show planktonic foraminiferaδ18O records9and (c) the green circles show the Bermuda Rise231Pa/230Th records from core OCE326-GGC5 (ref.9) for reference. (d) The blue diamonds show the diatom:coccolith ratios from biomarkers5from the East Equatorial Pacific. (e) The solid triangles show the Th-normalized opal accumulation rates from the Southern Ocean4, and the red dotted line shows the EPICA pCO2in parts per million by volume (p.p.m.v.) record from Antarctica63. These records indicate a widespread increase in diatom production and silicon utilization as a result of an increase in wind-driven upwelling and an increase in thermocline Si(OH)4concentrations. All error bars show ±2σs.d. The grey shaded box shows the opal-rich layer of HU890838-8PC; stronger utilization is shown by the darker shading. Figure 3: Results from sediment core HU89038-8PC. ( a ) Silicon isotope results from sediment core HU89038-8PC (error bars show ±2 σ s.d.). The solid squares show δ 30 Si of Ethmodiscus rex diatoms; the hollow squares show δ 30 Si of Spumellarian radiolarians; the grey squares show δ 30 Si of >63 μm opal. There is a positive correlation between the E. rex and radiolarian δ 30 Si measurements (Pearson’s correlation coefficient R =+0.71, n =10, P =0.02). The >63 μm opal δ 30 Si matched the E. rex opal δ 30 Si from the same depth within error, which would be expected, given that E. rex constituted over 95% of the bulk opal. The lines show calculated utilization of Si by the E. rex (solid line) and radiolarian (dashed line) cells, using a fractionation factor of −1.1‰ for the E. rex . We plot the mean utilization calculated for radiolarians with fractionation factors ranging from −0.9 to −2.1‰ (Methods). ( b ) The cyan circles show planktonic foraminifera δ 18 O records [9] and ( c ) the green circles show the Bermuda Rise 231 Pa/ 230 Th records from core OCE326-GGC5 (ref. 9 ) for reference. ( d ) The blue diamonds show the diatom:coccolith ratios from biomarkers [5] from the East Equatorial Pacific. ( e ) The solid triangles show the Th-normalized opal accumulation rates from the Southern Ocean [4] , and the red dotted line shows the EPICA pCO 2 in parts per million by volume (p.p.m.v.) record from Antarctica [63] . These records indicate a widespread increase in diatom production and silicon utilization as a result of an increase in wind-driven upwelling and an increase in thermocline Si(OH) 4 concentrations. All error bars show ±2 σ s.d. The grey shaded box shows the opal-rich layer of HU890838-8PC; stronger utilization is shown by the darker shading. Full size image We quantified this system further using a simple fractionation model (see Methods), feeding E. rex with Si(OH) 4 from thermocline waters assuming an open system [29] and a fractionation factor of −1.1‰ (ref. 20 ). The remaining Si(OH) 4 not utilized by the E. rex was then supplied to the radiolarians, which fractionate Si in an isotopically closed system. The calculated utilization does not change significantly when the assumed fractionation factor for radiolarians is varied within reasonable boundaries. From our model, we deduce that at the beginning of HS1, E. rex utilized a negligible proportion of the Si(OH) 4 available, suggesting some other factor limited production, and the radiolarians utilized ~40%. By 17 ka, the E. rex and radiolarians were utilizing up to 50 and 100% of the Si(OH) 4 available to them, respectively ( Fig. 3 ), suggesting total Si(OH) 4 utilization. Such large and rapid changes in utilization exceeded any deglacial change in Si utilization in the Southern Ocean or Eastern Equatorial Pacific upwelling zones [31] , [32] , and are indicative of significant changes in upwelling and mixing at the inception of HS1. We can use the simple Si isotope fractionation model (after ref. 22 ) to provide quantitative limits on the opal production and export rates during the utilization peak of the HS1 diatom event. Today, the Si(OH) 4 concentrations of subthermocline waters in the North Atlantic are ~15–20 μM, and mix into the subsurface waters to provide ~1.5 μM Si (ref. 1 ). Our sponge spicule δ 30 Si results from KNR140-2-56GGC indicate that 30 μM Si were available for biological uptake in subthermocline during HS1, suggesting subsurface waters would have a concentration of ~2–3 μM Si assuming similar advection and diffusion rates as today. For an upwelling water supply rate of 1 m −2 per day [33] , our calculations suggests that ~20 mmol Si m −2 per day were utilized during this time period, although it is possible that there were variations in Si(OH) 4 concentration of subthermocline waters that have not been detected by our sponge spicule record ( Fig. 2 ). Assuming 50% of the opal is recycled in the subsurface (the global average [34] ), we estimate a total of ~10 mmol Si m −2 per day was exported to the deep ocean at the inception of HS1, compared with ~1.3 mmol Si m −2 per day today in a Mode-Water eddy driven bloom [35] . A more sophisticated two-box biogeochemical model achieves similar opal output fluxes (see Methods, Supplementary Figs 4 and 5 ). The assemblage composition and isotopic signals from the diatoms and radiolarians indicate an environmental setting in which upwelling Si(OH) 4 -rich waters are utilized at depths greater than 100 m by E. rex with radiolarians (and small diatoms) taking up the isotopically enriched Si(OH) 4 ‘leftovers’. How could such a scenario evolve? E. rex require strong stratification to dominate ecosystems, with a breakdown in stratification triggering sinking and sedimentation [21] . It is possible that the enhanced Si(OH) 4 concentrations within the thermocline that occurred as a result of changes in ocean circulation at the inception of HS1 (17.5–18 ka) could have promoted the growth of giant diatom species such as E. rex , in a similar way to the modern North Pacific. The frequent replenishment of nutrients resulted in low Si utilization. Rapid sinking and sedimentation of the E. rex cells would then have been caused by deep mixing, which could have been caused by enhanced wind stress as observed for other HS pre-30 ka (ref. 36 ), turbulent mixing due to icebergs or upwelling at an unstable oceanic front [37] . A review of core descriptions reveals that the occurrence of E. rex during the deglacial appears to be limited to a region of ~100–200 km diameter near the Bermuda Rise ( Supplementary Fig. 6 ) that could be indicative of a mesoscale forcing mechanism, concentrating the cells into a particular region rather than a large-scale shift in frontal systems. Today, wind-driven mesoscale processes are known to extend to at least 1,000 m depth [38] , bringing up deep sources of nutrients and driving phytoplankton blooms that are as strong as the spring blooms driven by seasonal wind-driven deep mixing ( Fig. 1 ). In particular, Mode-Water eddies are known to drive changes in ecology, promoting large diatom production in the Sargasso Sea for example, Chaetoceros [35] . Rapid sinking and sedimentation of the E. rex cells could therefore have been triggered during early HS1 by periodic eddy processes, due to wind or iceberg forcing, which would also have replenished nutrient supplies to the subsurface. By 17 ka, a progressive increase in stratification may have led to higher Si utilization in surface waters, as a result of meltwater, reduced wind stress or frontal zone convergence. In the Sargasso Sea, stratification is unlikely to have resulted from a reduction in wind stress during HS1 (ref. 36 ) or from the convergence of frontal systems. Introduction of meltwater lenses during ice-rafting events from the North are consistent with records of smaller diatoms [7] and the deposition of ice-rafted debris at the Bermuda Rise [9] , and the onset of changes in the planktonic foraminiferal δ 18 O record from HU89038-PC8 ( Fig. 3 ). The high percentage counts of the deep-dwelling radiolarian Cycladophora davisiana Ehrenberg observed near the top of the section indicate that periodic and intense upwelling still occurred, albeit at a lower frequency, replenishing the nutrient supply and promoting more occasional E. rex sinking and sedimentation. E. rex production continued until either stratification broke down or thermocline Si concentrations declined and a system similar to the modern was established. Comparing the results from the simple fractionation model to sedimentary opal accumulation rates from the Bermuda Rise shows that the increase in export of opal from the subsurface/thermocline to deep waters was greater than the increase in opal burial, indicating deep opal remineralization and a reduction in the burial efficiency ( Table 1 ). Low resolution data for a nearby core on the Bermuda Rise (GGC5 and WHOI long core CDH19 Henry, McManus et al. , unpublished data) indicate that the thorium-normalized Holocene sediment flux is ~2 g cm −2 ka −1 , of which 4–5% is opal, giving a sedimentary opal flux of <0.1 g SiO 2 cm −2 ka −1 . In contrast, the opal percentages at HS1 and the last glacial maximum (LGM) were ~6–8 and 4–6%, respectively, with HS1 and LGM thorium-normalized sediment accumulation rates of 3.7 g cm −2 ka −1 and 5.6 g cm −2 ka −1 , respectively, giving sedimentary opal fluxes of ~0.25 g SiO 2 cm −2 ka −1 for HS1 and 0.28 g SiO 2 cm −2 ka −1 for the LGM ( Table 2 ). The Holocene sedimentary opal flux equates to ~10 mmol Si m −2 per year, which represents a preservation efficiency of ~20% of the observed sinking flux of 50 mmol Si m −2 per year of opal from surface to deep waters [1] . This estimated HS1 sedimentary opal flux is more than double that of the Holocene or modern. The greater abundance of E. rex in the diatom assemblage did not appear to markedly increase the opal flux to the sediments at HS1 compared with the preceding LGM. However, observations and modelling of the modern ocean indicate that in regions where large diatoms grow, the increase in export due to rapid sinking of material out of the surface ocean is accompanied by an increase in deep remineralization [39] . The HS1 sedimentary opal flux equates to ~40 mmol Si m −2 per year, which—depending on the assumed length of the bloom (~30 days)—is consistent with a lower preservation efficiency of ~10–15% of the opal exported out of surface waters from our model simulations (that is, total preservation efficiency of ~5–10%). As the order of magnitude increase in overall sediment accumulation rates at that time should have strongly enhanced the preservation potential of opal deposited on the seafloor, it appears likely that greater dissolution occurred in the mid-depth to deep ocean. This dissolution may have had an influence on the assemblage of opal fossils preserved, although smaller diatoms and delicate radiolarians are still present in the opal-rich layer of HU089038. Table 1 Summary of sinking opal and sedimentary opal fluxes and indication of preservation efficiency . Full size table Table 2 A comparison of HS1 and LGM opal burial in the Sargasso Sea (unpublished data from Henry, McManus et al . ). Full size table High export of opal into deep waters would have been accompanied by an increase in carbon export (see Methods). E. rex are also found from a similar time in a nearby core OCE326-5GGC during a period of relatively low 230 Th-normalized carbonate flux, indicating diatom productivity was promoted without a relative increase in productivity of carbonate producers [9] . This shift towards opal producers relative to carbonate-secreting phytoplankton would have resulted in at least a localized change in ocean alkalinity acting to further drawdown CO 2 in the near-surface waters [40] . Palaeoceanographic records show that, during the deglacial, there were widespread pulses of diatom production, which we suggest were due to the abrupt breakdown of stratification, similar to—but to a greater extent than—today, as a result of different wind-driven mechanisms linked by atmospheric teleconnections, which supplied nutrients to large regions of the surface ocean rather than slow diffusion processes [4] , [5] , [6] , [31] , [41] . The E. rex pulse studied here either occurs at a similar time as, or at the inception of, increased diatom accumulation throughout Atlantic upwelling regions (for example, Northwest Atlantic [6] , [8] , [42] ). This upwelling, together with an increase in thermocline Si(OH) 4 concentration, stimulated widespread diatom productivity and enhanced Si utilization ( Fig. 3 ). These wind-driven processes in the low latitudes of the Atlantic and Pacific appeared to occur approximately concurrently and early in HS1 (refs 5 , 14 , 43 ) at the onset of the significant changes in upwelling that occurred in the Southern Ocean ( Fig. 3 ). Assuming these offsets are real, and not a result of uncertainties in the age models, they could highlight the importance of not only global changes in preformed nutrients but also more localized processes that allow these preformed nutrients to reach the surface, which drove ecological regime shifts and marine carbon uptake. The early upwelling signal in some regions of the low latitudes, at the onset of the significant changes in upwelling that occurred in the Southern Ocean ( Fig. 3 ), suggests climatic changes in the North Atlantic were transferred to the Southern hemisphere via atmospheric and oceanic teleconnections, at the same time as the initiation of the pCO 2 rise recorded in ice cores ( Fig. 3 ). Despite such high biological productivity, physical changes in ocean circulation and subsequent release of stored carbon overwhelmed any biological response, associated with a rise in pCO 2 (ref. 4 ). Silicon isotope measurements Sponge spicules were hand-picked from the sand-sized fraction (>63 μm) of core KNR140-2-56GGC and cleaned according to ref. 23 . For HU89038-8PC, the opal fraction of the ~300–500 cm section was removed from the sand fraction, which constitutes a relatively small proportion of the sediment, using flotation [19] . These biogenic opal fractions were cleaned initially using a filtration method adapted from ref. 44 . In brief, the samples were suspended in deionized water and poured into a cylindrical filter funnel, fitted with a 200-μ filter mesh at the base, which was clamped into a water bath. The whole apparatus was placed in an ultrasonic bath and sonicated for at least half an hour, flushing through the sample with at least 1 l of deionized water. This method removes the smaller grains of pyrite and removes particles adhered to the opal leaving a clean biogenic component. The filter mesh was removed from the apparatus, and the different biogenic components were hand-picked: (1) large Spumellaria radiolarians (dominated by relatively shallow dwelling forms, see below); and (2) a monospecific sample of E. rex fragments. Smear slides were made of the >63 μ fraction for radiolarian counts and species identification. The different biogenic opal components were rinsed in 18 MΩ Milli-Q water, dried down in Teflon vials, and then dried down again in distilled concentrated HNO 3 at 180 °C. While still hot, 500 μl of 0.4 M NaOH were added to each sample and dissolved over 1 day (in the case of E. rex samples) or 3 days (in the case of the radiolarians and sponges) at 100 °C. The samples were acidified using 0.2 N in-house Teflon-distilled HCl and purified using cation exchange resin according to ref. 45 . The samples were analysed for silicon isotope composition using the Neptune multi-collector inductively coupled plasma mass spectrometer at the WHOI plasma facility. Mass bias and matrix effects were corrected using internal Mg-doping according to ref. 46 . The results are reported as δ 30 Si values related to the standard NBS28. Repeat measurements were carried out for all the samples (typically n =3, depending on sample size) and the mean isotope ratio was calculated in each case. Long-term external reproducibility was assessed by measuring the δ 30 Si of a biogenic opal standard [47] over several months. The reproducibility of the mean δ 30 Si (−3.43‰) from the repeat measurements of the standard each run using the Mg-doping method was ±0.1‰ (2 s.d.). The repeat measurements carried out for the samples also generally agreed within ±0.1‰ or better. A three-isotope plot ( δ 29 Si versus δ 30 Si) of all of the opal samples measured in this study fall on a straight line through the origin with a gradient of ~0.51, indicative of mass-dependent fractionation ( Supplementary Fig. 2 ). Two >63 μ opal fraction samples from HU89038-8PC [19] were measured to investigate the impact that the other siliceous species, in addition to E. rex , had on δ 30 Si. The samples were heated in H 2 O 2 (30%), dried and then fused with NaOH pellets in silver crucibles at 730 °C for 10 min. The fusion cake was cooled briefly, and then quenched in 18 MΩ cm Milli-Q water, left overnight and acidified with 2 N in-house Teflon-distilled HCl. The solutions were purified by cation exchange resin as above and measured for silicon isotopes by multi-collector inductively coupled plasma mass spectrometer without Mg correction (external reproducibility ~0.16‰ for δ 30 Si (ref. 47 ). By preparing these samples using a different method, we can show there is no analytical bias introduced through choice of sample dissolution process. Radiocarbon measurements The age model for KNR140-2-56GGC was based on existing planktonic foraminiferal radiocarbon measurements and an additional five radiocarbon measurements ( Supplementary Table 2 ) of Globigerinoides ruber (white) picked (greater than 150 μm size fraction) measured at the National Ocean Sciences Accelerator Mass Spectrometry facility at Woods Hole Oceanographic Institution. Calendar ages were calculated using Calib v. 6.1.0, using Marine09, using a reservoir age of 525 years, and a Δ R of 148 (±70). The age model for HU089038-8PC was based on radiocarbon measurements obtained from ref. 19 . Radiolarian depth of habitat Most polysystine radiolarians live in water depths of less than 250 m and this is especially true for the Spumellarians (spherical shelled species) [48] , [49] . The specimens analysed in this study are large (>100 μm), frequently spongy, Spumellarians. The large spongy species belong to the genera Spongechinus , Spongodrymus and Plegmosphaera . Spongodrymus and other large spongy Spumellarians often have associated with them symbiotic algae (zooxanthellae) [50] . For these symbionts to thrive, the host radiolarians must spend some time within the euphotic zone. The most common radiolarian in the assemblage, Actinomma medianum (Haeckel), has been recovered from water depths of less than 100 m in the eastern Pacific [51] . Other Spumellarians include Acanthosphaera actinota (Haeckel), which was raised from less than 100 m in numerous plankton samples from the California Current System [51] , A. arcadophorum (Haeckel) and a species of Hexacontium probably, H. axatrias (Haeckel), reported by ref. 52 , together with the former two, from the shallowest (389 m) of a series of sediment traps moored in the western equatorial Atlantic. Although precise depth ranges for the radiolarian species analysed in this study are not known, the information available suggests that most, if not all, of the large Spumellarians analysed spent most of their lives in waters shallower than 250 m and possibly less than 100 m. Calculating utilization Utilization was calculated for the E. rex and radiolarians assuming open fractionation [29] : where f =utilization, δ opal =silicon isotope composition of the opal, δ Si(OH)4 =the silicon isotope composition of the input seawater (assumed to be +1.6 per mil for either North Atlantic or AAIW [53] ) and ε =fractionation by opal-producing organisms (assumed to be −1.1 per mil). The Si isotopic composition of AAIW was assumed to be constant during this period because of a lack of significant change in diatom δ 30 Si from the subAntarctic during this period [54] . The remaining seawater composition was calculated according to equation (2): HS1 biogeochemical model A simple box model of biogeochemical cycling in the Sargasso Sea was created using Stella (version 9.1) based on the schematic shown in Supplementary Fig. 4 . Details of the variables used are in Supplementary Table 3 (refs 55 , 56 ). The model comprises two boxes, an intermediate box (below 100 m water depth) inhabited by diatoms and a shallow box (0–100 m water depth) inhabited by radiolarians. The intermediate box is connected to an input from underlying thermocline waters. The intermediate and shallow boxes are linked by diffusive and advective pathways according to the water column structure. The shallow box can additionally lose water through lateral transfer. To simplify the model, no lateral transfer is assumed for the intermediate box. For any box i of volume V i , change in concentration ( C i ) is equal to the difference in the flux ( F ) in and the flux out of Si. An initial state of strong stratification exists and no initial Si is available in either box. Thermocline waters have a concentration of 30 μM Si. At t =0, diffusion and advection is turned on between the thermocline and the two boxes. Flux by diapycnal diffusion (across isopycnals), F vd , is modelled assuming the isopycnals are nearly horizontal (equation (3)). Eddy diffusive mixing (along sloping isopyncals) is assumed to be negligible. Advection is dominated by large-scale Ekman pumping, with the possibility of ageostrophic flow [33] , [57] . Where K d is the diapycnal turbulent diffusion coefficient and z is depth. E. rex is allowed to grow in the intermediate box, and radiolarians are allowed to grow in the surface box, with Si utilization constrained with the silicon isotope data from core HU89038-8PC. Fractionation of Si isotopes is calculated for each organism according to equations (1) and (2). Opal flux ( φ ) is given by equation (4) and depends on the utilization ( f ), the amount of Si available ( C i ) and the proportion of opal that undergoes dissolution (1- P ). Carbon fluxes are calculated assuming Si:C~0.13 mol/mol (ref. 58 ). The impact of isotopic fractionation [59] during dissolution was tested (percentage dissolution based on ref. 60 ). The silica flux was sensitive to the advective flux ( Supplementary Fig. 5A ) but was not sensitive to dissolution ( Supplementary Fig. 5B ). The fractionation factor for E. rex was allowed to vary between −0.9 and −2.1‰; the fractionation factor for Spumellaria radiolarians was allowed to vary between −1.1 and −2.1‰. Total silica flux and concentration was not sensitive to the fractionation factors used. Surface utilization was sensitive to the fractionation factors selected ( Supplementary Fig. 5C ). Our estimate of mean daily sinking opal flux during the utilization peak of HS1 from the model is the same order of magnitude as the total annual flux driven by modern winter convection today. The increased supply is due to a combination of intense stratification, punctuated by mesoscale processes and the widespread increase in thermocline Si(OH) 4 concentrations resulting from the enhanced contribution of southern component water to the North Atlantic. The increase in diatom production would also have led to an increase in the carbon export production, and so CO 2 drawdown, to deep waters. For a typical Si:C molar ratio of 0.13 (ref. 58 ), the model gives a total carbon flux of ~15 g C m −2 per day. For E. rex growing over the period of 1 month, and with a high export efficiency typical of diatom-dominated ecosystems, this sinking could result in carbon export to deep waters of ~300–400 g C m −2 per year during HS1, which is over an order of magnitude greater than the export in the Sargasso Sea today [58] (~10 g C m −2 per year). How to cite this article: Hendry, K. R. et al. Silicon isotopes indicate enhanced carbon export efficiency in the North Atlantic during deglaciation. Nat. Commun. 5:3107 doi: 10.1038/ncomms4107 (2014).